Dynamic information routing in complex networks Flexible information routing fundamentally underlies the function of many biological and artificial networks. Yet, how such systems may specifically communicate and dynamically route information is not well understood. Here we identify a generic mechanism to route information on top of collective dynamical reference states in complex networks. Switching between collective dynamics induces flexible reorganization of information sharing and routing patterns, as quantified by delayed mutual information and transfer entropy measures between activities of a network’s units. We demonstrate the power of this mechanism specifically for oscillatory dynamics and analyse how individual unit properties, the network topology and external inputs co-act to systematically organize information routing. For multi-scale, modular architectures, we resolve routing patterns at all levels. Interestingly, local interventions within one sub-network may remotely determine nonlocal network-wide communication. These results help understanding and designing information routing patterns across systems where collective dynamics co-occurs with a communication function. Attuned function of many biological or technological networks relies on the precise yet dynamic communication between their subsystems. For instance, the behaviour of cells depends on the coordinated information transfer within gene-regulatory networks [1] , [2] and flexible integration of information is conveyed by the activity of several neural populations during brain function [3] . Identifying general mechanisms for the routing of information across complex networks thus constitutes a key theoretical challenge with applications across fields, from systems biology to the engineering of smart distributed technology [4] , [5] , [6] . Complex systems with a communication function often show characteristic dynamics, such as oscillatory or synchronous collective dynamics with a stochastic component [7] , [8] , [9] , [10] , [11] . Information is carried in the presence of these dynamics within and between neural circuits [12] , [13] , living cells [14] , [15] , ecological or social groups [16] , [17] as well as technical communication systems, such as ad hoc sensor networks [18] , [19] . While such dynamics could simply reflect the properties of the interacting unit's, emergent collective dynamical states in biological networks can actually contribute to the system's function. For example, it has been hypothesized that the widely observed oscillatory phenomena in biological networks enable emergent and flexible information routing [12] . Yet, what are the precise mechanism by which collective dynamics contribute to organizing communication in networks? Moreover, how do the intrinsic dynamics of units, their interaction topology and function as well as external driving signals and noise create specific patterns of information routing? In this article, we derive a theory for information routing in complex networked systems, revealing the joint impact of all these elements. We identify a generic mechanism to dynamically route information in complex networked systems by conveying information in fluctuations around a collective dynamical reference state. Propagation of information then depends on the underlying reference dynamics and switching between multiple stable states induces flexible rerouting of information, even if the physical network stays unchanged. For oscillatory dynamics, analytic predictions show precisely how the physical coupling structure, the units’ properties and the dynamical state of the network co-act to generate a specific communication pattern, quantified by time-delayed mutual information (dMI) [20] , [21] and transfer entropy [22] curves between time-series of the network’s units. Resorting to a collective phase description [23] , our theory further resolves communication patterns at all levels of multi-scale, modular topologies [24] , [25] , as ubiquitous, for example, in the brain connectome and biochemical regulatory networks [26] , [27] , [28] , [29] . Interestingly, local interventions within one sub-network may remotely modify information transfer between other seemingly unrelated sub-networks. Finally, a combinatorial number of information routing patterns (IRPs) emerge if several multi-stable subsystems are combined into a larger modular network. These relations between multi-scale connectivity, collective network dynamics and flexible information routing have potential applications in the reconstruction and design of gene-regulatory circuits [15] , [30] , wireless communication networks [4] , [19] or to the analysis of cognitive functions [31] , [32] , [33] , [34] , [35] , among others. Moreover, these results offer generic insights into mechanisms for flexible and self-organized information routing in complex networked systems. Information routing via collective dynamics To better understand how collective dynamics may contribute to specifically distribute bits of information from external or locally computed signals through a network or to it s downstream components we first consider a generic stochastic dynamical system. It evolves in time t according to where x =( x 1 ,…, x N ) denotes the variables of the network nodes, f describes the intrinsic dynamics of the network. The key premise is that the information to be routed through the network is carried in the stochastic external input ξ =( ξ 1 ,…, ξ N ) driving instantaneous state variable fluctuations. To access the role of collective dynamics in routing this information we consider a deterministic intrinsic reference state x (ref) ( t ) solving (2) in the absence of signals ( ξ =0). We use information theoretic measures that quantify the amount of information shared and transferred between nodes, independent of how this information is encoded or decoded. More precisely, we measure information sharing between signal x i ( t ) and the time d lagged signal x j ( t + d ) of nodes i and j in the network via the time-delayed mutual information (dMI) [20] , [21] Here p i ( t ) is the probability distribution of the variable x i ( t ) of unit i at time t and p i , j ( d ) ( t ) the joint distribution of x i ( t ) and the variable x j ( t + d ) lagged by d . As a second measure, we use the delayed transfer entropy (dTE) [22] (cf. Methods) that genuinely measures information transfer between pairs of units [36] . Asymmetries in the curves dMI i , j ( d ) and dTE i → j ( d ) then indicate the dominant direction in which information is shared or transferred between nodes (cf. Supplementary Note 1 ). To identify the role of the underlying reference dynamical state x (ref) ( t ) for network communication a small-noise expansion in the signals ξ turns a out to be ideally suited: while this expansion limits the analysis to the vicinity of a specific reference state which is usually regarded as a weakness of this technique, in the context of our study, this property is highly advantageous as it directly conditions the calculations on a particular dynamical state and enables us to extract it s role for the emergent pattern of information routing within the network. For white noise sources ξ this method yields general expressions for the conditional probabilities p ( x ( t + d )| x ( t )) that depend on x (ref) ( t ). Using this result the expressions for the dMI (2) and dTE (7) dMI i , j ( d ) and dTE i → j ( d ) become a function of the underlying collective reference dynamical state (cf. Methods and Supplementary Note 2 ). The dependency on this reference state then provides a generic mechanism to change communication in networks by manipulation the underlying collective dynamics. In the following we show how this general principle gives rise to a variety of mechanisms to flexibly change information routing in networks. We focus on oscillatory phenomena widely observed in networks with a communication function [32] , [34] , [35] , [37] , [38] . Information exchange in phase signals Oscillatory synchronization and phase locking [8] , [10] provide a natural way for the temporal coordination between communicating units. Key variables in oscillator systems are the phases φ i ( t ) at time t of the individual units i . In fact, a wide range of oscillating systems display similar phase dynamics [8] , [11] (cf. Supplementary Note 3 ) and phase-based encoding schemes are common, for example, in the brain [32] , [34] , [35] , genetic circuits [37] and artificial systems [38] . We first focus on systems in a stationary state with a stationary distribution for which the expressions for the dMI and dTE become independent of the starting time t and only depend on the lag d and reference state φ (ref) ( t ). To assess the dominant direction of the shared information between two nodes, we quantify asymmetries in the dMI curve by using the difference δ MI i , j =MI i → j −MI j → j between the integrated mutual informations and MI j → i . If this is positive, information is shared predominantly from unit i to j , while negative values indicate the opposite direction. Analogously, we compute the differences in dTE as δ TE i , j (cf. Methods and Supplementary Note 1 ). The set of pairs { δ MI i , j } or { δ TE i , j } for all i , j then capture strength and directionality of information routing in the network akin to a functional connectivity analysis in neuroscience [39] . We refer to them as IRPs. A range of networks of oscillatory units, with disparate physical interactions, connection topologies and external input signals support multiple IRPs. For instance, in a model of a gene-regulatory network with two oscillatory sub-networks ( Fig. 1a ) dMI analysis reveals IRPs with different dominant directions ( Fig. 1b–d , upper versus lower). The change is triggered by adding an external factor that degrades the transcribed mRNA in one of the oscillators and thereby changes its intrinsic frequency (see Methods). More complex changes in IRPs emerge in larger networks, possibly with modular architecture. In a network of interacting neuronal populations ( Fig. 1e ), different initial conditions lead to different underlying collective dynamical states. Switching between them induces complicated but specific changes in the IRPs ( Fig. 1f–h ). Different IRPs also emerge by changing a small number of connections in larger networks. Fig. 1i–l illustrates this for a generic system of coupled oscillators each close to a Hopf bifurcation. 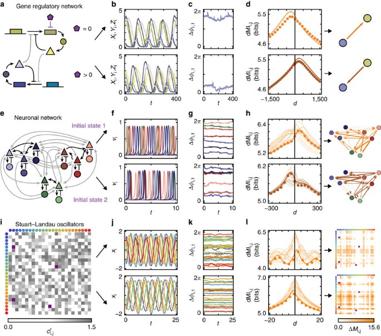Figure 1: Flexible information routing across networks. (a) Simple model of a gene-regulatory network of two coupled biochemical oscillators of Goodwin type (yellow and blue). An additional molecule (purple) degrades the transcribed mRNA in one of the oscillators and thereby changes its intrinsic frequency. Coupling strengths are gray coded (darker colour indicates stronger coupling), sharp arrows indicate activating and blunt arrows inhibiting influences (cf. Methods). (b) Stochastic oscillatory dynamics of the concentrations of the systems componentsxi(mRNA),yi(enzyme), andzi(protein),i∈{1, 2}. (c) Fluctuations of the phases extracted from the full dynamics relative to a reference unit. (d) dMI (dMI1,2) between the phase signals. The numerical data (dots) agrees well with the theoretical prediction (4) (solid lines). The asymmetry in the dMI curves aroundd=0 indicates a directed information sharing pattern summarized in the graphs (right). Arrow thickness indicates the strength of directed information sharing ΔMIi,jmeasured by the positively rectified differences of the areas below the dMIi,j(d) curve ford<0 andd>0. (e–h) Same as ina–dbut for a modular network of coupled neuronal sub-populations consisting each of excitatory (triangle) and inhibitory (disk) populations (Wilson–Cowan-type dynamics) that undergo neuronal oscillatory activity (cf. Methods). For the same network two different collective dynamical states accessed by different initial conditions give rise to two different information sharing patterns (f–htop versus bottom). (f) Oscillatory activitiesviof theN=8 excitatory populationsi. (i–l) As ina–dbut for generic oscillators close to a Hopf bifurcation (Stuart–Landau oscillators) each described by two-dimensional normal-form coordinates (xi,yi) connected to a larger network ofN=25 oscillators with coupling coefficientsci,jr(cf. Methods). Iniandl, connectivity matrices are shown instead of graphs. Two different network-wide IRPs arise (top versus bottom inj–l) by changing a small number of connection weights (purple entries iniandl). Figure 1: Flexible information routing across networks. ( a ) Simple model of a gene-regulatory network of two coupled biochemical oscillators of Goodwin type (yellow and blue). An additional molecule (purple) degrades the transcribed mRNA in one of the oscillators and thereby changes its intrinsic frequency. Coupling strengths are gray coded (darker colour indicates stronger coupling), sharp arrows indicate activating and blunt arrows inhibiting influences (cf. Methods). ( b ) Stochastic oscillatory dynamics of the concentrations of the systems components x i (mRNA), y i (enzyme), and z i (protein), i ∈ {1, 2}. ( c ) Fluctuations of the phases extracted from the full dynamics relative to a reference unit. ( d ) dMI (dMI 1,2 ) between the phase signals. The numerical data (dots) agrees well with the theoretical prediction (4) (solid lines). The asymmetry in the dMI curves around d =0 indicates a directed information sharing pattern summarized in the graphs (right). Arrow thickness indicates the strength of directed information sharing ΔMI i , j measured by the positively rectified differences of the areas below the dMI i , j ( d ) curve for d <0 and d >0. ( e – h ) Same as in a – d but for a modular network of coupled neuronal sub-populations consisting each of excitatory (triangle) and inhibitory (disk) populations (Wilson–Cowan-type dynamics) that undergo neuronal oscillatory activity (cf. Methods). For the same network two different collective dynamical states accessed by different initial conditions give rise to two different information sharing patterns ( f – h top versus bottom). ( f ) Oscillatory activities v i of the N =8 excitatory populations i . ( i – l ) As in a – d but for generic oscillators close to a Hopf bifurcation (Stuart–Landau oscillators) each described by two-dimensional normal-form coordinates ( x i , y i ) connected to a larger network of N =25 oscillators with coupling coefficients c i,j r (cf. Methods). In i and l , connectivity matrices are shown instead of graphs. Two different network-wide IRPs arise (top versus bottom in j – l ) by changing a small number of connection weights (purple entries in i and l ). Full size image In general, several qualitatively different options for modifying network-wide IRPs exist, all of which are relevant in natural and artificial systems: (i) changing the intrinsic properties of individual units (Fig. 1a–d); (ii) modifying the system connectivity ( Fig. 1i–l ); and (iii) selecting distinct dynamical states of structurally the same system ( Fig. 1e–h ). Theory of phase information routing To reveal how different IRPs arise and how they depend on the network properties and dynamics, we derive analytic expressions for the dMI and dTE between all pairs of oscillators in a network. We determine the phase of each oscillator i in isolation by extending its phase description to the full basin of attraction of the stable limit cycle [8] , [40] . For weak coupling, the effective phase evolution becomes where ω i is the intrinsic oscillation frequencies of node i and the coupling functions γ i , j (·) depend on the phase differences only. The final sum in (3) models external signals as independent Gaussian white noise processes ξ k and a covariance matrix i , k . The precise forms of γ i , j (·) and i , k generally depend on the specific system ( Supplementary Note 3 ). As visible from Fig. 1e–h , the IRP strongly depends on the underlying collective dynamical state. We therefore decompose the dynamics into a deterministic reference part and a fluctuating component . We focus on phase-locked configurations for the deterministic dynamics with constant phase offsets . We estimate the stochastic part via a small-noise expansion (Methods and Supplementary Note 4 , Theorem 1) yielding a first-order approximation for the joint probabilities p i , j ( d ) . Using (2) together with the periodicity of the phase variables, we obtain the dMI between phase signals in coupled oscillatory networks; here, I n ( k ) is the n th modified Bessel function of the first kind, and k i , j ( d ) is the inverse variance of a von Mises distributions ansatz for p i , j ( d ) . The system’s parameter dependencies, including different inputs, local unit dynamics, coupling functions and interaction topologies are contained in k i , j ( d ) . By similar calculations we obtain analytical expressions for dTE i → j (Methods and Supplementary Note 4 , Theorem 2). Our theoretical predictions well match the numerical estimates ( Fig. 1d,h,l , see also Fig. 2c,d below and Supplementary Figs 1 and 2 ). For independent input signals ( i , k =0 for i k ) we typically obtain similar IRPs determined either by the dMI or the transfer entropy ( Supplementary Fig. 1 ). Further, the results remain valid qualitatively when the noise level increases ( Supplementary Fig. 2 ). 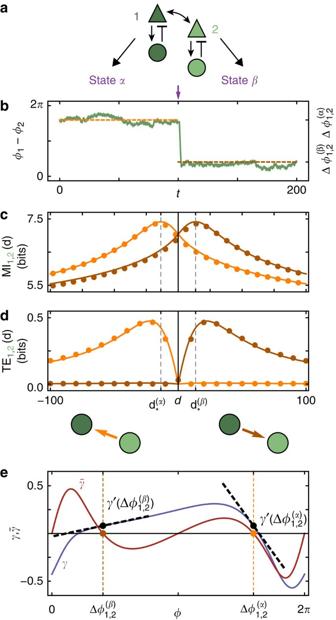Figure 2: Multi-stable dynamics and anisotropic information routing. (a) Two identical and symmetrically coupled neuronal circuits of Wilson–Cowan-type (dark and light green, modular sub-network inFig. 1e). The noise free (that is, input free) network displays two different stable oscillatory dynamical statesαandβ. (b) Phase difference Δφ1,2(t):=φ1(t)−φ2(t) between the extracted phases of the two neuronal populations is fluctuating around a locked valueof a the stable collective state α of the deterministic system (orange); a strong external perturbation (purple arrow) induces a switch to stochastic dynamics around the second stable deterministic reference stateβ(brown) with phase difference. (c) Delayed mutual information dMI1,2and (d) transfer entropy dTE1→2curves between the phase signals in statesα(orange) andβ(brown) for numerical data (dots) and theory (lines) as a function of the time delaydbetween the stochastic phase signalsφ1(t) andφ2(t+d). The change in peak latencies formtoin the dMI1,2curves and the asymmetry of the dTE1→2curves show anisotropic information routing for the two different states. Switching between the two dynamical states reverses the effective information routing pattern (IRP) (graphs, bottom). (e) Phase coupling functionγ(Δφ)=γ1,2(Δφ)=γ2,1(Δφ) (blue) between the two neuronal oscillators and its anti-symmetric part(red). The two zeros ofwith negative slope indicate the stable deterministic equilibrium phase differencesandof the dynamical statesαandβ, receptively. The directionality in the IRP arises due to symmetry breaking in the dynamics reflected in the different slopes ofγ(Δφ) (dashed lines): In the stateα, oscillator 1 receives inputs from oscillator 2 proportional to, while oscillator 2 is coupled to 1 proportional toin linear small-noise approximation (cf. equation (5)). Asis large deviations from the phase-locked state of oscillator 2 due to the noise inputs are strongly propagated to oscillator 1 to restore the phase-locking. Information injected to oscillator 2 is thus transmitted to oscillator 1. In contrast, inputs to oscillator 1 only weakly impact oscillator 2 asis small. In total, the information is thus dominantly routed from 2 to 1. Switching to the dynamical stateβreverses the roles of the oscillators and thus also the directionality of the information routing motive. Figure 2: Multi-stable dynamics and anisotropic information routing. ( a ) Two identical and symmetrically coupled neuronal circuits of Wilson–Cowan-type (dark and light green, modular sub-network in Fig. 1e ). The noise free (that is, input free) network displays two different stable oscillatory dynamical states α and β . ( b ) Phase difference Δ φ 1,2 ( t ):= φ 1 ( t )− φ 2 ( t ) between the extracted phases of the two neuronal populations is fluctuating around a locked value of a the stable collective state α of the deterministic system (orange); a strong external perturbation (purple arrow) induces a switch to stochastic dynamics around the second stable deterministic reference state β (brown) with phase difference . ( c ) Delayed mutual information dMI 1,2 and ( d ) transfer entropy dTE 1→2 curves between the phase signals in states α (orange) and β (brown) for numerical data (dots) and theory (lines) as a function of the time delay d between the stochastic phase signals φ 1 ( t ) and φ 2 ( t + d ). The change in peak latencies form to in the dMI 1,2 curves and the asymmetry of the dTE 1→2 curves show anisotropic information routing for the two different states. Switching between the two dynamical states reverses the effective information routing pattern (IRP) (graphs, bottom). ( e ) Phase coupling function γ (Δ φ )= γ 1,2 (Δ φ )= γ 2,1 (Δ φ ) (blue) between the two neuronal oscillators and its anti-symmetric part (red). The two zeros of with negative slope indicate the stable deterministic equilibrium phase differences and of the dynamical states α and β , receptively. The directionality in the IRP arises due to symmetry breaking in the dynamics reflected in the different slopes of γ (Δ φ ) (dashed lines): In the state α , oscillator 1 receives inputs from oscillator 2 proportional to , while oscillator 2 is coupled to 1 proportional to in linear small-noise approximation (cf. equation (5)). As is large deviations from the phase-locked state of oscillator 2 due to the noise inputs are strongly propagated to oscillator 1 to restore the phase-locking. Information injected to oscillator 2 is thus transmitted to oscillator 1. In contrast, inputs to oscillator 1 only weakly impact oscillator 2 as is small. In total, the information is thus dominantly routed from 2 to 1. Switching to the dynamical state β reverses the roles of the oscillators and thus also the directionality of the information routing motive. Full size image Mechanism of anisotropic information routing To better understand how a collective state gives rise to a specific routing pattern with directed information sharing and transfer, consider a network of two symmetrically coupled identical neural population models ( Fig. 2a ). Because of permutation symmetry, the coupling functions γ i , j , obtained from the phase reduction of the original Wilson–Cowan-type equations [41] (Methods, Supplementary Note 3 ), are identical. For biologically plausible parameters this network in the noiseless-limit has two stable phase-locked reference states ( α and β ). The fixed phase differences and are determined by the zeros of the anti-symmetric coupling with negative slope ( Fig. 2e ). For a given level of (sufficiently weak) noise, the system shows fluctuations around either one of these states ( Fig. 2b ) each giving rise to a different IRP. Sufficiently strong external signals can trigger state switching and thereby effectively invert the dominant communication direction visible from the dMI ( Fig. 2c ) and even more pronounced from the dTE ( Fig. 2d ) without changing any structural properties of the network. The anisotropy in information transfer in the fully symmetric network is due to symmetry broken dynamical states. For independent noise inputs, i , k = i δ i , k , that are moreover small, the evolution of , i ∈ {1,2}, near the reference state α reduces to with coupling constants , (Methods). As ( Fig. 2e ), the phase essentially freely fluctuates driven by the noise input 2 ξ 2 . This causes the system to deviate from the equilibrium phase difference . At the same time, the strongly negative coupling dominates over the noise term 1 ξ 1 and unit 1 is driven to restore the phase difference by reducing . Thus, is effectively enslaved to track and information is routed from unit 2 to 1, reflected in the dMI and dTE curves. The same mechanism accounts for the reversed anisotropy in communication when the system is near state β as the roles of units 1 and 2 are exchanged. Calculating the peak of the dMI curve in this example also provides a time scale at which maximal information sharing is observed (Methods, equation (10), see also Supplementary Note 4 ). It furthermore becomes clear that the directionality of the information transfer in general need not be related to the order in which the oscillators phase-lock because the phase-advanced oscillator can either effectively pull the lagging one, or, as in this example, the lagging oscillator can push the leading one to restore the equilibrium phase-difference. In summary, effective interactions local in state space and controlled by the underlying reference state together with the noise characteristics determine the IRPs of the network. Symmetry broken dynamical states then induce anisotropic and switchable routing patterns without the need to change the physical network structure. Information routing in networks of networks For networks with modular interaction topology [24] , [25] , [26] , [27] , [28] , our theory relating topology, collective dynamics and IRPs between individual units can be generalized to predict routing between entire modules. Assuming that each sub-network X in the noiseless limit has a stable phase-locked reference state, a second-phase reduction [23] generalized to stochastic dynamics characterizes each module by a single meta-oscillator with collective phase Φ X and frequency Ω X , driven by effective noise sources Ξ X with covariances Σ X , Y . The collective phase dynamics of a network with M modules then satisfies where Γ X , Y are the effective inter-community couplings ( Supplementary Note 5 ). The structure of equation (6) is formally identical to equation (3) so that the expressions for inter-node information routing (dMI i , j and dTE i → j ) can be lifted to expressions on the inter-community level (dMI X , Y and dTE X→Y ) by replacing node- with community-related quantities (that is, ω i with Ω X or γ ik with Γ X , K and so on; Supplementary Note 5 , Corollaries 3 and 4). Importantly, this process can be further iterated to networks of networks and so on. 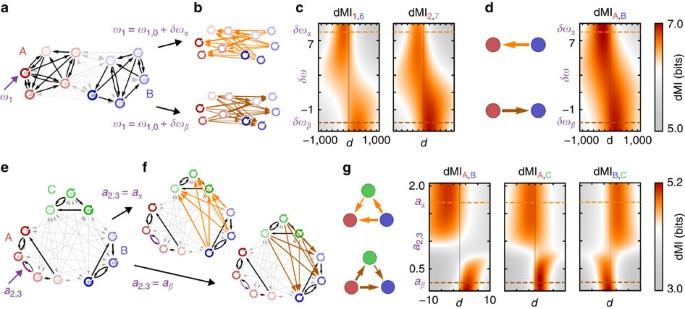Figure 3: Remotely induced rerouting of information in modular networks. (a) Network with two coupled communitiesAandB(red and blue) of oscillators close to a Hopf bifurcation. Changing the intrinsic frequency of a single nodei=1 fromω1+δωαtoω1+δωβinduces a collective reorganization of equilibrium phase differences, that result inboppositely directed information sharing patterns between the individual nodes of the two modules (top versus bottom). (c) dMI between two pairs of nodes from the two different clusters as a function of the time delaydand frequency changeδω1of oscillator 1. The change of the peak from positive to negative delays reflecting the inversion of the information routing is visible. (d) Information routing patterns (IRPs) calculated from the hierarchically reduced system for the two configurations inb(left) and as a function ofδω1(right) reflect the inversion on the finer scale (b,c). (e) Hierarchical network of three coupled modules of phase oscillators. (f) A change in the connection strengtha2,3fromaαtoaβbetween two nodes (3A→2A) in sub-networkAinduces an inversion of information routing direction between the remote sub-networksBandC. (g) Full IRPs calculated form the hierarchical reduced system fora2,3=aαanda2,3=aα(left) and as a function ofa2,3for all pairs of modules (density plots, right). The transition is not continuous but rather switch like. Figure 3 shows examples of information flow patterns resolved at two scales. The information routing direction on the larger scale reflects the majority and relative strengths of IRPs on the finer scale. Figure 3: Remotely induced rerouting of information in modular networks. ( a ) Network with two coupled communities A and B (red and blue) of oscillators close to a Hopf bifurcation. Changing the intrinsic frequency of a single node i =1 from ω 1 + δω α to ω 1 + δω β induces a collective reorganization of equilibrium phase differences, that result in b oppositely directed information sharing patterns between the individual nodes of the two modules (top versus bottom). ( c ) dMI between two pairs of nodes from the two different clusters as a function of the time delay d and frequency change δω 1 of oscillator 1. The change of the peak from positive to negative delays reflecting the inversion of the information routing is visible. ( d ) Information routing patterns (IRPs) calculated from the hierarchically reduced system for the two configurations in b (left) and as a function of δω 1 (right) reflect the inversion on the finer scale ( b , c ). ( e ) Hierarchical network of three coupled modules of phase oscillators. ( f ) A change in the connection strength a 2,3 from a α to a β between two nodes (3 A →2 A ) in sub-network A induces an inversion of information routing direction between the remote sub-networks B and C . ( g ) Full IRPs calculated form the hierarchical reduced system for a 2,3 = a α and a 2,3 = a α (left) and as a function of a 2,3 for all pairs of modules (density plots, right). The transition is not continuous but rather switch like. Full size image Nonlocal information rerouting via local interventions The collective quantities in the system (6) are intricate functions of the network properties at the lower scales. Intriguingly, the coupling functions Γ X , Y not only depend on the nonlocal interactions between units i X of module X and j Y of cluster Y but also on purely local properties of the individual clusters. In particular, the form of Γ X , Y is a function of the intrinsic local dynamical states and of both clusters as well as the phase response Z X of sub-network X (see Methods and Supplementary Note 5 ). Thus IRPs on the entire network level depend on local community properties. This establishes several generic mechanisms to globally change information routing in networks via local changes of modular properties, local connectivity or via switching of local dynamical states. In a network consisting of two sub-networks ( Fig. 3a ) the local change of the frequency of a single Hopf-oscillator in sub-network A induces a nonlocal inversion of the information routing between cluster A and B ( Fig. 3b–d ). In Fig. 3e–f , the direction in which information is routed between two sub-networks B and C of coupled phase oscillators is remotely changed by increasing the strength of a local link in module A . The origin in both examples is a non-trivial combination of several factors: the (small) manipulations alter the collective cluster frequency Ω A and the local dynamical state which in turn changes the collective phase response Z A and the effective noise strength Ξ A of cluster A . These changes all contribute to changes in the effective couplings Γ X , Y as well as in the inter-cluster phase-locking values ΔΦ X , Y =Φ X −Φ Y (cf. Supplementary Note 5 and Supplementary Fig. 3 ). The changes in these properties, which enter the expressions for the information sharing and routing measures ( Fig. 2 and Supplementary Note 4 ) then cause the observed changes in information routing direction. Interestingly, the transition in information routing has a switch-like dependency on the changed parameter ( Fig. 3c,d,g ) promoting digital like changes of communication modes. Combinatorially many information routing patterns. Combinatorial many information routing patterns As an alternative to interventions on local properties, also switching between multi-stable local dynamical states can induce global information rerouting. In the example in Fig. 4 , each of the M =3 modules X ∈ { A , B , C } exhibits alternative phase-locked states (labelled α X and β X , Supplementary Section 6 and Supplementary Fig. 4 ). For sufficiently weak coupling, this local multi-stability is preserved in the dynamics of the entire modular network. Consequently each choice of the possible combinations of ‘local’ states gives rise to at least one network-wide collective state. Certain combinations of local states can give rise to one or even multiple globally phase-locked states (for example, [ α A β B α C ] in Fig. 4 ). Others support non-phase-locked dynamics that gives rise to time-dependent IRPs (cf. Fig. 4c and below). Thus, varying local dynamical states in a hierarchical network flexibly produces a combinatorial number of different IRPs in the same physical network. 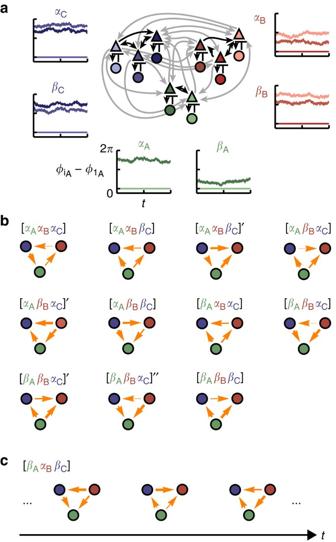Figure 4: Combinatorially many IRPs in networks with locally multi-stable dynamics. (a) Modular circuit as inFig. 1e. Without inter-module coupling (grey arrows), each of theM=3 communitiesX∈{A,B,C} exhibits multi-stability between two phase-locked configurations, denoted as statesαXandβX(insets). The characteristics of these states remain present in the full network once weak coupling between the modules is introduced. We refer to these states as local dynamical states. (b) Information routing patterns (IRPs) between the hierarchically reduced sub-networks for different combinations of the local dynamical states,that give rise to globally phase-locked dynamics. Arrows between nodesXandYindicate strength (line width) and sign (arrow direction) of the information routing quantified via the difference in integrated dTE curves between the nodes (see Methods). The same combination of local dynamical states () can give rise to more than one globally phase-locked collective state marked with dashes, i.e.,,…. each giving rise to a separate IRP: For fixed local dynamical states the global network is multi-stable and choosing between those components is changing the information routing similarly as inFig. 2. (c) The local dynamical state configuration [βAαBβC] generates a periodic global dynamical state (cf.Supplementary Fig. 3) in which the hierarchically reduced IRP (graphs) becomes time-dependent (cf. alsoSupplementary Note 6). Figure 4: Combinatorially many IRPs in networks with locally multi-stable dynamics. ( a ) Modular circuit as in Fig. 1e . Without inter-module coupling (grey arrows), each of the M =3 communities X ∈ { A , B , C } exhibits multi-stability between two phase-locked configurations, denoted as states α X and β X (insets). The characteristics of these states remain present in the full network once weak coupling between the modules is introduced. We refer to these states as local dynamical states . ( b ) Information routing patterns (IRPs) between the hierarchically reduced sub-networks for different combinations of the local dynamical states , that give rise to globally phase-locked dynamics. Arrows between nodes X and Y indicate strength (line width) and sign (arrow direction) of the information routing quantified via the difference in integrated dTE curves between the nodes (see Methods). The same combination of local dynamical states ( ) can give rise to more than one globally phase-locked collective state marked with dashes, i.e. , ,…. each giving rise to a separate IRP: For fixed local dynamical states the global network is multi-stable and choosing between those components is changing the information routing similarly as in Fig. 2 . ( c ) The local dynamical state configuration [ β A α B β C ] generates a periodic global dynamical state (cf. Supplementary Fig. 3 ) in which the hierarchically reduced IRP (graphs) becomes time-dependent (cf. also Supplementary Note 6 ). Full size image Time-dependent information routing General reference states, including periodic or transient dynamics, are not stationary and hence the expressions for the dMI and dTE become dependent on the time t . For example, Fig. 4c shows IRPs that undergo cyclic changes due to an underlying periodic reference state (cf. also Supplementary Note 6 and Supplementary Fig. 5a-c ). In systems with a global fixed point, systematic displacements to different starting positions in state space give rise to different stochastic transients with different and time-dependent IRPs ( Supplementary Fig. 5d ). Similarly, switching dynamics along heteroclinic orbits constitute another way of generating specific progressions of reference dynamics. Thus information ‘surfing’ on top of non-stationary reference dynamical configurations naturally yield temporally structured sequences of IRPs, resolvable also by other measures of instantaneous information flow [36] , [42] , [43] . The above results establish a theoretical basis for the emergence of information routing capabilities in complex networks when signals are communicated on top of collective reference states. We show how information sharing (dMI) and transfer (dTE) emerge through the joint action of local unit features, global interaction topology and choice of the collective dynamical state. We find that IRPs self-organize according to general principles (cf. Figs 2 , 3 , 4 ) and can thus be systematically manipulated. Employing formal identity of our approach at every scale in oscillatory modular networks (equations (3) versus (6), ) we identify local paradigms that are capable of regulating information routing at the nonlocal level across the whole network ( Figs 3 and 4 ). In contrast to self-organized technological routing protocols where local nodes use local routing information to locally propagate signals, such as in peer-to-peer networks [44] , in the mechanism studied here the information routing modality is set by the entire network’s collective dynamics. This collective reference state typically evolves on a slower timescale than the information carrying fluctuations that surf on top of it and is thus different from signal propagation in cascades [45] or avalanches [46] that dominate on shorter time scales. We derived theoretical results based on information sharing and transfer obtained via delayed mutual information and transfer entropy curves. Using these abstract measures our results are independent of any particular implementation of a communication protocol and thus generically demonstrate how collective dynamics can have a functional role in information routing. For example, in the network in Fig. 2 externally injected streams of information are automatically encoded in fluctuations of the rotation frequency of the individual oscillators. The injected signals are then transmitted through the network and decodable from the fluctuating phase velocity of a target unit precisely along those pathways predicted by the current state-dependent IRP ( Supplementary Note 7 and Supplementary Figs 6 and 7 ). Our theory is based on a small-noise approximation that conditions the analysis onto a specific underlying dynamical state. In this way, we extracted the precise role of such a reference state for the network’s information routing abilities. For larger signal amplitudes or in highly recurrent networks, in which higher order interactions can play an important role the expansion can be carried out systematically to higher orders using diagrammatic approaches [47] or numerically to accounting for better accuracy and non-Gaussian correlations (cf. also Supplementary Note 4 ). In systems with multi-stable states two signal types need to be discriminated: those that encode the information to be routed and those that indicate a switch in the reference dynamics and consequently the IRPs. If the second type of stimuli is amplified appropriately a switch between multi-stable states can be induced that moves the network into the appropriate IRP state for the signals that follow. For example, in the network of Fig. 2a switch from states α to β can be induced by a strong positive pulse to oscillator 2 (and vice versa). If such pulses are part of the input a switch to the appropriate IRP state will automatically be triggered and the network auto-regulates its IRP function ( Supplementary Fig. 6 ). More generally a separate part of the network that effectively filters out relevant signatures indicating the need for a different IRP could provide such pulses. Using the fact that local interventions are capable to switch IRPs in the network also the outcomes of local computations can be used to trigger changes in the global information routing and thereby enable context-dependent processing in a self-organized way. When information surfs on top of dynamical reference states the control of IRPs is shifted towards controlling collective network dynamics making methods from control theory of dynamical systems available to the control of information routing. For example, changing the interaction function in coupled oscillators systems [18] or providing control signals to a subset of nodes [48] , [49] are capable of manipulating the network dynamics. Moreover, switch-like changes (cf. Fig. 3 ) can be triggered by crossing bifurcation points and the control of IRPs then gets linked to bifurcation theory of network dynamical systems. While the mathematical part of our analysis focused on phase signals, including additional amplitude degrees of freedom into the theoretical framework can help to explore neural or cell signalling codes that simultaneously use activity- and phase-based representations to convey information [50] . Moreover, separating IRP generation, for example, via phase configurations, from actual information transfer, for instance in amplitude degrees of freedom, might be useful for the design of systems with a flexible communication function. The role of self-organized collective dynamics in information routing in biological systems is still speculative. Our theoretical study, identifying natural mechanisms for state-dependent sharing and transfer of information, may thus foster further experimental explorations that seek for conclusive proofs and exploring the nonlocal effects of local system manipulations. While recent experimental studies point towards functional roles of collective dynamics [31] , [35] , [51] , [52] , [53] , [54] the predicted phenomena, including nonlocal changes of information routing by local interventions, could be directly experimentally verified using methods available to date, such as synthetic patterned neuronal cultures [55] , electrochemical arrays [18] or synthetic gene-regulatory networks [5] ( Supplementary Note 8 ). In addition, our results are applicable to the inverse problem: Unknown network characteristics may be inferred by fitting theoretically expected dMI and dTE patterns to experimentally observed data. For example, inferring state-dependent coupling strengths could further the analysis of neuronal dynamics during context-dependent processing [33] , [35] , [39] , [53] , [54] , [56] . Modifying inputs, initial conditions or system-intrinsic properties may well be viable in many biological and artificial systems whose function requires particular information routing. For instance, on long time scales, evolutionary pressure may select a particular IRP by biasing a particular collective state in gene-regulatory and cell-signalling networks [2] , [15] , [57] ; on intermediate time scales, local changes in neuronal responses due to adaptation or varying synaptic coupling strength during learning processes [13] can impact information routing paths in entire neuronal circuits; on fast time scales, defined control inputs to biological networks or engineered communication systems that switch the underlying collective state, can dynamically modulate IRPs without any physical change to the network. Transfer entropy The dTE [22] from a time-series x i ( t ) to a time-series x j ( t ) is defined as with joint probability p i , j , j ( d ) = p ( x j ( t + d ), x i ( t ), x j ( t )) and p j , j ( d ) = p ( x j ( t + d ), x j ( t )). This expression is not invariant under permutation of i and j , implying the directionality of TE. For a more direct comparison with dMI in Fig. 2 , we define dTE i,j ( d ) by dTE i → j ( d ) for d >0 and by dTE j → i (− d ) for d <0 (cf. Supplementary Note 1 for additional details). Dynamic information routing via dynamical states For a dynamical system (2) the reference deterministic solution x (ref) ( t + s ) starting at x ( t ) is given by the deterministic flow x (ref) ( t + s )= F (ref) ( x ( t ), s ). The small-noise approximation for white noise ξ yields where denotes the normal distribution with mean x and covariance matrix Σ , and G ( s , x )= Df ( F ( x , s )). We assumed G ( s , x ) G ( t , x )= G ( t , x ) G ( s , x ). From this and the initial distribution p ( x ( t )), the dMI and transfer entropy dMI i , j ( d , t ) and dTE i → j ( d , t ) are obtained via (2) and (7). The result depends on time t , lag d and the reference state x (ref) (cf. Supplementary Note 2 for additional details). Oscillator networks In Fig. 1a , we consider a network of two coupled biochemical Goodwin oscillators [14] , [58] . Oscillations in the expression levels of the molecular products arise because of a nonlinear repressive feedback loop in successive transcription, translation and catalytic reactions. The oscillators are coupled via mutual repression of the translation process [59] . In addition, in one oscillator changes in concentration of an external enzyme regulate the speed of degradation of mRNAs, thus affecting the translation reaction, and, ultimately, the oscillation frequency. In Figs 1e , 2 and 4 we consider networks of Wilson–Cowan-type neural masses (population signals) [41] . Each neural mass intrinsically oscillates because of antagonistic interactions between local excitatory and inhibitory populations. Different neural masses interact, within and between communities, via excitatory synapses. In the generic networks in Figs 1i and 3a each unit is modelled by the normal form of a Hopf-bifurcation in the oscillatory regime together with linear coupling. Finally, the modular networks analysed in Fig. 3a,b are directly cast as phase-reduced models with freely chosen coupling functions. See the Supplementary Note 8 and Supplementary Figs 4, 8 and 9 for additional details, model equations and parameters and phase estimation. Analytic derivation of the dMI and dTE curves In the small-noise expansion [60] , both dMI and dTE curves have an analytic approximation: For stochastic fluctuations around some phase-locked collective state with constant reference phase offsets Δ φ i,j = φ i − φ j the phases evolve as in the deterministic limit, where Ω= ω i + k γ i , k (Δ φ i , k ) is the collective network frequency and the γ i,j (·) are the coupling functions from equation (3). In presence of noise, the phase dynamics have stochastic components . In first-order approximation, independent noise inputs i,j = i δ i,j yield coupled Ornstein–Uhlenbeck processes with linearized, state-dependent couplings given by the Laplacian matrix entries g i , j =− γ ′ i , j (Δ φ i , j ) and . The analytic solution to the stochastic equation (9) provides an estimate of the probability distributions, p i , p i , j ( d ) and p i , j , j ( d ) . Via (2) this results in a prediction for dMI i , j ( d ), equation (4), as a function of the matrix elements k i , j ( d ) specifying the inverse variance of a von Mises distribution ansatz for p i , j ( d ) . Similarly via (7) an expression for dTE i → j ( d ) is obtained. For the dependency of , and dTE i → j ( d ) on network parameters and further details, see the derivation of the theorems 1 and 2 in Supplementary Note 4 . Time scale for information sharing For a network of two oscillators as in Fig. (2) with linearized coupling strengths and and , maximizing dMI 1,2 ( d ) (see Supplementary Note 4 for full analytic expressions of dMI and dTE in two oscillator networks) yields Collective phase reduction Suppose that each node i = i X belongs to a specific network module X out of M ≤ N non-overlapping modules of a network. Then equation (3) can be simplified to equation (6) under the assumption that in the absence of noise every community X has a stable internally phase-locked state , where are constant phase offsets of individual nodes i X . Every community can then be regarded as a single meta-oscillator with a collective phase Φ X ( t ) and a collective frequency . The vector components of the collective phase response Z X , the effective couplings Γ X , Y and the noise parameters Σ X , Y and Ξ X are obtained through collective phase reduction and depend on the respective quantities ( ) on the single-unit scale (see Supplementary Note 5 for a full derivation). How to cite this article : Kirst, C. et al . Dynamic information routing in complex networks. Nat. Commun. 7:11061 doi: 10.1038/ncomms11061 (2016).